Decoding tumour phenotype by noninvasive imaging using a quantitative radiomics approach Human cancers exhibit strong phenotypic differences that can be visualized noninvasively by medical imaging. Radiomics refers to the comprehensive quantification of tumour phenotypes by applying a large number of quantitative image features. Here we present a radiomic analysis of 440 features quantifying tumour image intensity, shape and texture, which are extracted from computed tomography data of 1,019 patients with lung or head-and-neck cancer. We find that a large number of radiomic features have prognostic power in independent data sets of lung and head-and-neck cancer patients, many of which were not identified as significant before. Radiogenomics analysis reveals that a prognostic radiomic signature, capturing intratumour heterogeneity, is associated with underlying gene-expression patterns. These data suggest that radiomics identifies a general prognostic phenotype existing in both lung and head-and-neck cancer. This may have a clinical impact as imaging is routinely used in clinical practice, providing an unprecedented opportunity to improve decision-support in cancer treatment at low cost. Medical imaging is one of the major factors that have informed medical science and treatment. By assessing the characteristics of human tissue noninvasively, imaging is often used in clinical practice for oncologic diagnosis and treatment guidance [1] , [2] , [3] . A key goal of imaging is ‘personalized medicine’, where treatment is increasingly tailored on the basis of specific characteristics of the patient and their disease [4] . Much of the discussion of personalized medicine has focused on molecular characterization using genomic and proteomic technologies. However, as tumours are spatially and temporally heterogeneous, these techniques are limited. They require biopsies or invasive surgeries to extract and analyse what are generally small portions of tumour tissue, which do not allow for a complete characterization of the tumour. Imaging has great potential to guide therapy because it can provide a more comprehensive view of the entire tumour and it can be used on an ongoing basis to monitor the development and progression of the disease or its response to therapy. Further, imaging is noninvasive and is already often repeated during treatment in routine practice, on the contrary of genomics or proteomics, which are still challenging to implement into clinical routine. The most widely used imaging modality in oncology is X-ray computed tomography (CT), which assesses tissue density. Indeed, CT images of lung cancer tumours exhibit strong contrast reflecting differences in the intensity of a tumour on the image, intratumour texture and tumour shape ( Fig. 1a ). However, in clinical practice, tumour response to therapy is only measured using one- or two-dimensional descriptors of tumour size (RECIST and WHO, respectively) [5] . Although a change in tumour size can indicate response to therapy, it often does not predict overall or progression free survival [6] , [7] . Although some investigations have characterized the appearance of a tumour on CT images, these characteristics are typically described subjectively and qualitatively (‘moderate heterogeneity’, ‘highly spiculated’, ‘large necrotic core’). However, recent advances in image acquisition, standardization and image analysis allow for objective and precise quantitative imaging descriptors that could potentially be used as noninvasive prognostic or predictive biomarkers. 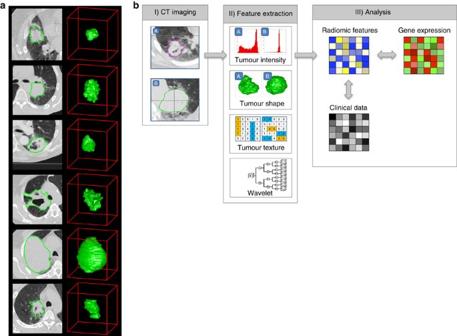Figure 1: Extracting radiomics data from images. (a) Tumours are different. Example computed tomography (CT) images of lung cancer patients. CT images with tumour contours left, three-dimensional visualizations right. Please note strong phenotypic differences that can be captured with routine CT imaging, such as intratumour heterogeneity and tumour shape. (b) Strategy for extracting radiomics data from images. (I) Experienced physicians contour the tumour areas on all CT slices. (II) Features are extracted from within the defined tumour contours on the CT images, quantifying tumour intensity, shape, texture and wavelet texture. (III) For the analysis the radiomics features are compared with clinical data and gene-expression data. Figure 1: Extracting radiomics data from images. ( a ) Tumours are different. Example computed tomography (CT) images of lung cancer patients. CT images with tumour contours left, three-dimensional visualizations right. Please note strong phenotypic differences that can be captured with routine CT imaging, such as intratumour heterogeneity and tumour shape. ( b ) Strategy for extracting radiomics data from images. (I) Experienced physicians contour the tumour areas on all CT slices. (II) Features are extracted from within the defined tumour contours on the CT images, quantifying tumour intensity, shape, texture and wavelet texture. (III) For the analysis the radiomics features are compared with clinical data and gene-expression data. Full size image Radiomics is an emerging field that converts imaging data into a high dimensional mineable feature space using a large number of automatically extracted data-characterization algorithms [8] , [9] . We hypothesize that these imaging features capture distinct phenotypic differences of tumours and may have prognostic power and thus clinical significance across different diseases. Here we assess the clinical relevance of 440 radiomic features, many of which currently have no known clinical significance, in seven independent cohorts consisting of 1,019 lung cancer and head-and-neck cancer patients. Two data sets are used to assess the stability of the features, four data sets to assess the prognostic value of radiomic features on lung cancer patients and head-and-neck cancer patients, and one data set for association with gene-expression profiles of lung cancer patients ( Fig. 2 ). Our results reveal that radiomics data contain strong prognostic information in both lung and head-and-neck cancer patients, and are associated with the underlying gene-expression patterns. These results suggest that radiomics decodes a general prognostic phenotype existing in multiple cancer types. Radiomics can have a large clinical impact, as imaging is used in routine practice worldwide, providing a method that can quantify and monitor phenotypic changes during treatment. 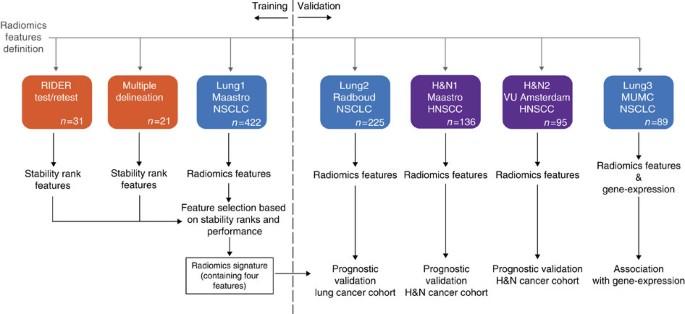Figure 2: Analysis workflow. The defined radiomic features algorithms were applied to seven different data sets. Two data sets were used to calculate the feature stability ranks, RIDER test/retest and multiple delineation respectively (both orange). The Lung1 data set, containing data of 422 non-small cell lung cancer (NSCLC) patients, was used as training data set. Lung2 (n=225), H&N1 (n=136) and H&N2 (n=95) were used as validation data sets. The Lung3 data set (n=89) was used for association of the radiomic signature with gene expression profiles. For the multivariate analysis, only one fixed four-feature radiomic signature was tested in the validation data sets. Figure 2: Analysis workflow. The defined radiomic features algorithms were applied to seven different data sets. Two data sets were used to calculate the feature stability ranks, RIDER test/retest and multiple delineation respectively (both orange). The Lung1 data set, containing data of 422 non-small cell lung cancer (NSCLC) patients, was used as training data set. Lung2 ( n =225), H&N1 ( n =136) and H&N2 ( n =95) were used as validation data sets. The Lung3 data set ( n =89) was used for association of the radiomic signature with gene expression profiles. For the multivariate analysis, only one fixed four-feature radiomic signature was tested in the validation data sets. Full size image Association of radiomic data with clinical data To assess the value of radiomic features to capture phenotypic differences of tumours, we performed an integrated analysis assessing prognostic performance and association with gene expression in lung and head-and-neck cancer data sets. First, we defined 440 quantitative image features describing tumour phenotype characteristics by: (I) tumour image intensity, (II) shape, (III) texture and (IV) multiscale wavelet ( Fig. 1b , Supplementary Methods ). To investigate radiomic expression patterns we extracted radiomic features from the Lung1 data set, consisting of 422 non-small cell lung cancer (NSCLC) patients ( Fig. 2 ). Unsupervised clustering revealed clusters of patients with similar radiomic expression patterns ( Fig. 3 ). We compared the three main clusters of patients with clinical parameters ( Fig. 3b ), and found significant association with primary tumour stage (T-stage; P <1 × 10 −20 , χ 2 test) and overall stage ( P =3.4 × 10 −3 , χ 2 test), wherein cluster I was associated with lower stages. N-stage (lymph node) and M-stage (metastasis), however, showed no correspondence with the radiomic expression patterns ( P =0.46 and P =0.73, respectively, χ 2 test). 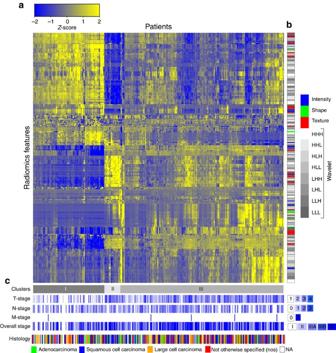Figure 3: Radiomics heat map. (a) Unsupervised clustering of lung cancer patients (Lung1 set,n=422) on theyaxis and radiomic feature expression (n=440) on thexaxis, revealed clusters of patients with similar radiomic expression patterns. (b) Clinical patient parameters for showing significant association of the radiomic expression patterns with primary tumour stage (T-stage;P<1 × 10−20,χ2test), overall stage (P=3.4 × 10−3,χ2test) and histology (P=0.019,χ2test). (c) Correspondence of radiomic feature groups with the clustered expression patterns. Figure 3: Radiomics heat map. ( a ) Unsupervised clustering of lung cancer patients (Lung1 set, n =422) on the y axis and radiomic feature expression ( n =440) on the x axis, revealed clusters of patients with similar radiomic expression patterns. ( b ) Clinical patient parameters for showing significant association of the radiomic expression patterns with primary tumour stage (T-stage; P <1 × 10 −20 , χ 2 test), overall stage ( P =3.4 × 10 −3 , χ 2 test) and histology ( P =0.019, χ 2 test). ( c ) Correspondence of radiomic feature groups with the clustered expression patterns. Full size image Furthermore, a significant association with histology ( P =0.019, χ 2 test) was observed, wherein squamous cell carcinoma showed a higher presence in cluster II. Looking at the representation of the feature groups ( Fig. 3c ), there was no correspondence between the feature group and radiomic expression patterns. Prognostic value of radiomic data The possible association of radiomic features with survival was then explored by Kaplan–Meier survival analysis. For training we used the Lung1 data set, and for validation the Lung2, H&N1, H&N2 data sets ( Fig. 2 ). The radiomic features were not normalized on any data set, and only the raw values were used that were directly computed from the DICOM images. To ensure a completely independent validation, the median value of each feature was computed on the training Lung1 data set, and locked for use as a threshold in the validation data sets to assess the survival differences without retraining. In Supplementary Fig. 1 we show Kaplan–Meier survival curves for four representative features. Features describing heterogeneity in the primary tumour were associated with worse survival in all four data sets. Also, patients with more compact/spherical tumours had better survival probability. Overall, the median threshold derived from Lung1 yielded a significant survival difference for 238 features (54% of total 440; G-rho test, false discovery rate (FDR) 10%) in the Lung2 validation data set. Furthermore, there was a significant survival difference for 135 features (31%) in H&N1 and for 186 features in H&N2 (42%). Sixty-six (15%) of the features derived from Lung1 were significant for survival in all three validation data sets (Lung2, H&N1 and H&N2). Building prognostic radiomic signature To build a prognostic radiomic signature, the analysis was divided in training and validation phases ( Fig. 2 ). For the training phase, we first explored feature stability determined in both test-retest and inter-observer setting. Using the publicly available RIDER [10] data set, consisting of 31 sets of test-retest CT scans that were acquired approximately 15 min apart, we tested how consistent the radiomic features were between the test and the retest scan. The multiple delineation data set, where five oncologists delineated lesions on CT scans from 21 patients [11] , was used to test the stability of the radiomic features to variation in manual delineations. For each feature, we compared the stability ranks for test-retest and multiple delineation with prognosis in the Lung1 training data set. Although the stability ranks did not use any information about prognosis, in general, features with higher stability for test-retest and delineation inaccuracies showed higher prognostic performance ( Supplementary Fig. 2 ). This is possibly due to reduced amount of noise in the stable features and supports the use of stability ranks for feature selection. To test the multivariate performance of a radiomic signature, we used the workflow depicted in Fig. 2 and Supplementary Fig. 3 . We focused our analysis on the 100 most stable features, which were determined by averaging the stability ranks of RIDER data set and multiple delineation data set. To remove redundancy within the radiomic information, we selected the single best performing radiomic feature from each of the four-feature groups, and combined these top four features into a multivariate Cox proportional hazards regression model for prediction of survival. The resulting radiomic signature consisted of (I) ‘Statistics Energy’ ( Supplementary Methods Feature 1) describing the overall density of the tumour volume, (II) ‘Shape Compactness’ (Feature 16) quantifying how compact the tumour shape is, (III) ‘Grey Level Nonuniformity’ (Feature 48) a measure for intratumour heterogeneity and (IV) wavelet ‘Grey Level Nonuniformity HLH’ (Feature Group 4), also describing intratumour heterogeneity after decomposing the image in mid-frequencies. The weights of each of the features in the signature were fitted on the training data set Lung1. Prognostic validation of radiomic signature The performance of the four-feature radiomic signature was validated in the data sets Lung2, H&N1 and H&N2 ( Fig. 2 ) using the concordance index (CI), which is a generalization of the area under the ROC curve [12] . The radiomic signature had good performance on the Lung2 data (CI=0.65, P =2.91 × 10 −09 , Wilcoxon test), and a high performance in H&N1 (CI=0.69, P =7.99 × 10 −07 , Wilcoxon test) and H&N2 (CI=0.69, P =3.53 × 10 −06 , Wilcoxon test). In Fig. 4a the Kaplan–Meier curves are shown. 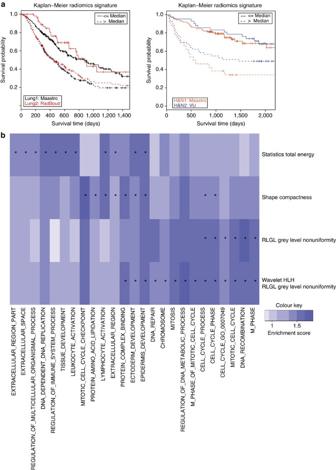Figure 4: Prognostic performance and gene-expression association of the radiomics signature. (a) Radiomic signature performance. Kaplan–Meier curves demonstrating performance of the radiomic signature on the lung cancer data sets (left) and the head-and-neck cancer data sets (right). The signature was built on the Lung1 data (n=422). The signature had a good performance in the Lung2 (CI=0.65,P=2.91 × 10−09, Wilcoxon test,n=225), and a high performance in H&N1 (CI=0.69,P=7.99 × 10−07, Wilcoxon test,n=136) and H&N2 (CI=0.69,P=3.53 × 10−06, Wilcoxon test,n=95) validation data sets. (b) Association of radiomic signature features and gene expression using gene-set enrichment analysis (GSEA) in the Lung3 data set (n=89). Gene sets that have been significantly enriched (FDR=20%) for at least one of the four radiomic features are indicated with an asterisk. The corresponding normalized enrichment scores (NES), GSEA’s primary statistic, for all radiomic signature features is displayed in a heat map, where light blue means low and dark blue means high NES. Figure 4: Prognostic performance and gene-expression association of the radiomics signature. ( a ) Radiomic signature performance. Kaplan–Meier curves demonstrating performance of the radiomic signature on the lung cancer data sets (left) and the head-and-neck cancer data sets (right). The signature was built on the Lung1 data ( n =422). The signature had a good performance in the Lung2 (CI=0.65, P =2.91 × 10 −09 , Wilcoxon test, n =225), and a high performance in H&N1 (CI=0.69, P =7.99 × 10 −07 , Wilcoxon test, n =136) and H&N2 (CI=0.69, P =3.53 × 10 −06 , Wilcoxon test, n =95) validation data sets. ( b ) Association of radiomic signature features and gene expression using gene-set enrichment analysis (GSEA) in the Lung3 data set ( n =89). Gene sets that have been significantly enriched (FDR=20%) for at least one of the four radiomic features are indicated with an asterisk. The corresponding normalized enrichment scores (NES), GSEA’s primary statistic, for all radiomic signature features is displayed in a heat map, where light blue means low and dark blue means high NES. Full size image Although volume had a good performance in all data sets, the radiomic signature performed significantly better, suggesting that radiomic features contain relevant, complementary information for prognosis ( Supplementary Table 1 ). Furthermore, combining the radiomic signature with volume was significantly better than volume alone in all data sets. Comparing the radiomic signature with the TNM staging [13] , we see that the signature performance was better in both Lung2 and H&N2 and comparable in H&N1 ( Supplementary Table 1 ). Importantly, combining the radiomic signature with TNM staging showed a significant improvement in all data sets, compared with TNM staging alone. Furthermore, we assessed if the radiomics signature preserved the significant prognostic performance compared with the treatment that the patients received. We found that the signature preserved its prognostic performance for all the treatment groups (radiation or concurrent chemoradiation), for both Lung and H&N cancer patients ( Supplementary Table 2 ), demonstrating the complementary value of radiomics for each treatment type. Human papillomavirus (HPV) is an important determinant in head-and-neck cancer patients, especially those with oropharyngeal carcinoma for prognosis and may guide future treatment selection. We did not find a significant association between radiomic signature prediction and HPV status in a combined analysis in the H&N1 and H&N2 data set ( P =0.17, Wilcoxon test, Supplementary Table 3 ). However, we found that the signature preserved its prognostic performance in the HPV-negative group (CI=0.66), consisting of the majority of patients (76%, n =130), demonstrating the complementary value of radiomics to HPV screening. To assess the association between the radiomic signature and the underlying biology, we compared the radiomic signature with gene-expression profiles (Lung3 data set, Fig. 2 ) using gene-set enrichment analysis (GSEA) [1] , [14] . We found significant associations between the signature features and gene-expression patterns ( Fig. 4b ). Further, the radiomic features are significantly associated with different biologic gene sets, demonstrating that radiomic features probe different biologic mechanisms. It is noteworthy that both intratumour heterogeneity features in the signature (Feature III and IV) were strongly correlated with cell cycling pathways, indicating an increased proliferation for more heterogeneous tumours. Medical imaging is one of the major factors informing medical science and treatment. Its potential resides in its ability to assess the characteristics of human tissue noninvasively, and therefore is routinely used in clinical practice for oncologic diagnosis and treatment guidance and monitoring. However, traditionally, medical imaging has been a subjective or qualitative science. Recent advances in medical imaging acquisition and analysis allow the high-throughput extraction of informative imaging features to quantify the differences that oncologic tissues exhibit in medical imaging. Radiomics applies advanced computational methodologies to medical imaging data to convert medical images into quantitative descriptors of oncologic tissues [8] . In this study, we analysed 440 radiomic features quantifying tumour phenotypic differences based on its image intensity, shape and texture. In a large data set of 1,019 lung and head-and-neck cancer patients, of which we extracted radiomic features on computed tomography images, we found that a large number of radiomic features have prognostic power, many of which their prognostic implication have not been described before. Furthermore, our integrated analysis showed that features selected on the basis of their stability and reproducibility were also the most informative features, which indicates the power of integrating independent data sets for radiomic feature selection and model building. We showed as well that a radiomic signature, capturing intratumour heterogeneity, was strongly prognostic and validated in three independent data sets of lung and head-and-neck cancer patients, and was associated with gene-expression profiles. To avoid any form of over-fitting or bias, we performed a robust statistical validation: only one radiomics signature (containing four radiomic features) was validated in data of 545 patients in independent validation data sets ( Fig. 2 and Supplementary Fig. 3 ). The four features were selected on the basis of feature stability and prognostic performance in the discovery data set only. The top performing feature ‘Grey Level Nonuniformity’ (Feature 48) and the most dominant features in the radiomic signature (Features III and IV), quantified intratumour heterogeneity. Indeed, it is often hypothesized that intratumour heterogeneity is exhibited on different spatial scales, for example at the radiological, macroscopic, cellular and the molecular (genetics) level. Radiological tumour phenotype characteristics may thus be useful to investigate the underlying evolving biology. It is known that multiple subclonal populations coexist within tumours, reflecting extensive intratumoral ‘somatic evolution’ [15] , [16] . This heterogeneity is a clear barrier to the goal of personalized therapy based on molecular biopsy-based assays, as the identified mutations and gene-expression does not always represent the entire population of tumour cells [17] , [18] . Radiomics circumvents this by assessing the comprehensive three-dimensional tumour bulk. The study presented here probes heterogeneity and demonstrates corresponding clinical importance in two cancer types. Furthermore, we demonstrated association of intratumour heterogeneity with proliferation, a general hallmark of cancer. Overall, the lung-derived radiomic signature had better performance in head and neck compared with lung cancer. One reason could be that head-and-neck images were acquired with head immobilization, whereas lung images were acquired with free breathing and are affected by patient movement or respiration, resulting in relatively more image noise. Nonetheless, our results show that the radiomic signature could be transferred from lung to head-and-neck cancer, which suggests that the signature identifies a general prognostic tumour phenotype. Our method provides a noninvasive (and therefore with no risk of infection or complications that accompany tissue biopsies), fast, low cost and repeatable way of investigating phenotypic information, potentially speeding up the development of personalized medicine. Furthermore, we show that the radiomic signature is significantly associated with the underlying gene-expression patterns, suggesting that inter-patient differences of gene expression are larger than intra-patient differences. The clinical impact of our results are illustrated by the fact that it advances knowledge in the analysis and characterization of tumours in medical images, previously not done, and provides knowledge currently not used in the clinic. We showed the complementary performance of radiomic features with TNM staging for prediction of outcome, which illustrates the clinical importance of our findings as TNM is routinely used in the clinic. Currently, the TNM staging system is used for risk stratification and treatment decision making. However, the TNM staging system is primarily based on resectability of the tumour, whereas a larger number of NSCLC patients will receive primary treatment with radiotherapy either alone or combined with chemotherapy. Therefore, the TNM staging system is insufficient for risk stratification of this group of patients, in particular to make the decision between curative treatment (concomitant radiochemotherapy) or palliative treatment especially in elderly patients, a growing issue in western countries. Our results show that the radiomics signature is performing better in independent cohorts than the TNM classification. In future clinical trials, this inexpensive method can be used as well for pretreatment risk stratification (for example, high, low risk). Furthermore, we have shown for the first time the translational capability of radiomics in two cancer types (lung and head-and-neck cancer). These results indicate that radiomics quantifies a general prognostic cancer phenotype that likely can broadly be applied to other cancer types. Similar observations have been made in gene-expression studies where signatures are prognostic across different diseases [19] . Analysis of image features applied to medical imaging has been a largely studied field and extensive literature exists. However, the majority of previous work describes the use of imaging features focused in the detection of small nodules in, for example, mammograms or chest CT/positron emission tomography (PET) scans, or in the differential diagnosis of malignant versus benign nodules (computed-aided diagnostics). However, applications and methodologies are distinct from our study. Quantitative imaging for personalized medicine is a recent field, with a limited number of publications [12] , [20] , [21] , [22] , [23] , [24] , [25] , [26] , [27] . The main clinical question of this research is not the diagnosis, but how to extract more useful information from the tumour phenotype that can be used for personalized medicine. Therefore, we assessed the association of radiomics with clinical factors, prognosis and gene-expression levels, using large amounts of features and with external and independent validation cohorts of patients. The most important message in our study is that there is prognostic and biologic information enclosed in routinely acquired CT imaging and was evident in two cancer types. It is known that variability in image acquisition exists across hospitals and that this is a reality in clinical practice. However, in our analysis we used data directly generated from the scanner and the features were calculated from the RAW imaging data, without any pre-processing or normalization. As there was no correction by cohort or scanner type, this illustrates the translational potential of our results and it is a strong argument in favour of a multicentric application of radiomics. The radiomics signature had strong prognostic power in these independent data sets generated in daily clinical practice. Furthermore, we expect that with better standardization and imaging protocols, the power of radiomics will even further improve. Among others, the quantitative imaging network of the National Institute of Health, as well as the quantitative imaging biomarker alliance, investigates future directions by performing phantom studies and discussing with vendor’s open and standardized protocols for image acquisition [2] , [3] . Due to the large availability of noninvasive imaging performed routinely in a large number of cancer patients and the automated feature algorithms, the results of this work could stimulate further research of image-based quantitative features. Also, we presented evidence that the defined radiomic feature-metrics are platform independent, though this should be studied further, and can potentially be applied to other image modalities, such as magnetic resonance imaging or PET. This approach can have a large impact as imaging is routinely used in clinical practice, worldwide, in all stages of diagnoses and treatment, providing an unprecedented opportunity to improve medical decision-support. Radiomics features We defined 440 radiomic image features that describe tumour characteristics and can be extracted in an automated way. The features can be divided into four groups: (I) tumour intensity, (II) shape, (III) texture and (IV) wavelet features. The first group quantified tumour intensity characteristics using first-order statistics, calculated from the histogram of all tumour voxel intensity values. Group 2 consists of features based on the shape of the tumour (for example, sphericity or compactness of the tumour). Group 3 consists of textual features that are able to quantify intratumour heterogeneity differences in the texture that is observable within the tumour volume. These features are calculated in all three-dimensional directions within the tumour volume, thereby taking the spatial location of each voxel compared with the surrounding voxels into account. Group 4 calculates the intensity and textural features from wavelet decompositions of the original image, thereby focusing the features on different frequency ranges within the tumour volume ( Supplementary Fig. 4 ). All feature algorithms were implemented in Matlab. In the Supplementary Methods , the feature algorithms are described. Data sets We applied a radiomic analysis to seven image data sets. An overview of the data sets is presented in Fig. 2 . All research was carried out in accordance with Dutch law. The Institutional Review Boards of each of the participating centres approved the studies: Lung1, Lung3, H&N1 (Maastricht University Medical Center (MUMC+), Maastricht, The Netherlands), Lung2 (Radboud University Medical Center (RUMC), Nijmegen, The Netherlands) and H&N2 (VU University Medical Center (VUMC), Amsterdam, The Netherlands). The Multiple delineation data set is publicly available (downloaded from: www.cancerdata.org ). This study was conducted according to national laws and guidelines and approved by the appropriate local trial committee at Maastricht University Medical Center (MUMC1), Maastricht, The Netherlands. The RIDER data set consists of 31 NSCLC patients with two CT scans acquired approximately 15 min apart [10] . We used this data set to assess stability of the features for test-retest. The multiple delineation data set consists of 21 NSCLC patients where the tumour volume was delineated manually on CT/PET scans by five independent oncologists [11] . We used this data set to assess stability of the features for delineation inaccuracies. The Lung1 data set consists of 422 NSCLC patients that were treated at MAASTRO Clinic, The Netherlands. For these patients, CT scans, manual delineations, clinical and survival data were available. We used this data set to assess the prognostic value of the radiomic features and to build a radiomic signature. The Lung2 data set consists of 225 NSCLC patients that were treated at Radboud University Nijmegen Medical Centre, The Netherlands. For these patients, CT scans, manual delineations, clinical and survival data were available. We used this data set to validate the prognostic value of the radiomic features and signature in an independent NSCLC cohort. The H&N1 data set consists of 136 head-and-neck squamous cell carcinoma (HNSCC) patients treated at MAASTRO Clinic, The Netherlands. For these patients, CT scans, manual delineations, clinical and survival data were available. We used this data set to validate the prognostic value of the radiomic features and signature in HNSCC patients. The H&N2 data set consists of 95 HNSCC patients treated at the VU University Medical Center Amsterdam, The Netherlands. For these patients, CT scans, manual delineations, clinical and survival data were available. We used this data set to validate the prognostic value of the radiomic features and signature in a second cohort of HNSCC patients. The Lung3 data set consists of 89 NSCLC patients that were treated at MAASTRO Clinic, The Netherlands. For these patients pretreatment CT scans, tumour delineations and gene expression profiles were available. We used this data set to associate imaging features with gene-expression profiles. In the Supplementary Methods and Supplementary Tables 4–7 , further descriptions of the data sets are presented. The discovery Lung1 data set, consisting of CT images for 422 NSCLC patients, and the Lung3 data set consisting of CT images and gene-expression profiling for 89 NSCLC patients, are publicly available at The Cancer Imaging Archive, Lung1: https://wiki.cancerimagingarchive.net/display/Public/NSCLC-Radiomics and Lung3: https://wiki.cancerimagingarchive.net/display/Public/NSCLC-Radiomics-Genomics , as well as on www.cancerdata.org . Sample size To reduce any form of over-fitting or bias in the multivariate analysis, we trained on data the Lung1 data sets ( n =422), selecting the features and fixing the weights, and tested only one signature (containing four features) in data of 545 patients in the independent validation data sets. There was no need for randomization as the patients originated from distinct groups. Patients were included in the analysis with the following criteria: confirmed primary tumour, patients underwent treatment with curative intent. Excluded from this analysis were patients receiving no or palliative treatment and patients with previous lung or head-and-neck cancer. Data analysis An overview of the analysis is shown in Fig. 2 . The analysis was divided in training and validation phases. For the training phase, we first explored feature stability determined in both test-retest and inter-observer setting. The RIDER and multiple delineation data sets were used to assess stability of the features to select the most informative features for further investigation. Using the RIDER test-retest data set, we tested the stability of the radiomic features between test and retest [10] . For each patient, we extracted the radiomic features from both scans. A stability rank was calculated for each feature, using the intraclass correlation coefficient, where a higher intraclass correlation coefficient rank corresponds to a more stable feature. We assessed the feature stability for delineation inaccuracies using a multiple delineation data set [11] . All radiomic features were computed for five delineations per patient, and a stability rank per feature was calculated using the Friedman test. The Friedman test is a nonparametric repeated measurement test for a non-Gaussian population. A rank of 1 indicated the most stable feature for delineation inaccuracies and 440 the least stable feature. All 440 radiomic features were extracted for the Lung1, Lung2, H&N1 and H&N2 data sets. The radiomic features were not normalized on any data set, and only the raw values were used that were directly computed from the DICOM image. To explore the association of the radiomics features with survival, we used Kaplan–Meier analysis in a training and validation phase. To ensure a completely independent validation, the median threshold of each feature on the Lung1 data set was computed, and then this threshold was used in the validation data sets (Lung2, H&N1 and H&N2) to split the survival curves. We used the G-rho rank test for censored survival data to test for significant differences between the two survival curves. P -values were corrected for multiple testing by controlling the FDR of 10%, the expected proportion of false discoveries amongst the rejected hypotheses. To assess the multivariate performance of radiomic features we built a signature. We selected the 100 most stable features, determined by averaging the stability ranks of RIDER data set and multiple delineation data set. Next, we computed the performance in the Lung 1 data set of each of the selected 100 features using the concordance index (CI) [12] . This measure is comparable with the area under the curve but can also be used for Cox regression analysis. From each of the four-feature groups, we selected the single best performing feature for prognosis in the Lung1 data set, and combined these top four features into a multivariate Cox proportional hazards regression model for prediction of survival. The weights of the model were fitted on the Lung1 data set. We applied the radiomic signature to the validation data sets Lung2, H&N1 and H&N2, and the performance was assessed with the CI. To calculate significance between two models we used a bootstrap approach, for 100 times we calculated the CI of both models from 100 randomly selected samples. The Wilcoxon test was used to assess significance. A similar approach was used to assess if the signature had significant power, compared with random (CI=0.5). We used a bootstrap approach, for 100 times we calculated the CI of the radiomics signature based on 100 randomly selected samples with correct outcome data, as well as on 100 randomly chosen samples with random outcome data. The Wilcoxon test was used to assess significance, between the two distributions. To assess the complementary effect of the signature with clinical parameters, we built a new model with the prediction of the signature as one input and the clinical parameter as the other input. The weight of the clinical parameter was fitted on the training data set Lung1. To assess the association of the radiomic signature with gene expression, we used the Lung3 data set. Gene expression of 89 patients was measured on Affymetrix chips with the custom chipset HuRSTA_2a520709 for 21,766 genes. Expression values were normalized with the RMA algorithm5 in the Affy package in Bioconductor. For each of the four features in the radiomic signature, we calculated the Spearman rank correlation to gene expression and used the corresponding P -values to obtain a rank of genes representing high-to-low agreement. Each of these gene ranks were used to perform a pre-ranked version of GSEA [14] on the C5 collection of MSigDB [28] , which contains gene sets associated with specific GO terms. We only regarded gene sets of size 15 to 500. Local FDRs were calculated on the normalized enrichment scores (NES), primary statistic of GSEA and only gene sets enriched with an FDR of ≤20% were retained. Figure 4b displays gene sets that have been significantly enriched (FDR ≤20%) for at least one of four radiomic features (indicated by an asterisk). The corresponding absolute NES in all of the four features are given color-coded, where light blue means low and dark blue means high NES. How to cite this article: Aerts, H. J. W. L. et al . Decoding tumour phenotype by noninvasive imaging using a quantitative radiomics approach. Nat. Commun. 5:4006 doi: 10.1038/ncomms5006 (2014).